Safe storage of radical initiators within a polyaromatic nanocapsule 2,2'-Azobisisobutyronitrile and its derivatives are standard reagents for polymer and organic syntheses that generate radical species on stimuli by light or heat. Radical initiators like the azo compounds are unstable so that they should be kept in the dark at low temperature to avoid photochemical and thermal decomposition as well as accidental explosion. Here we report the spontaneous and quantitative encapsulation of the radical initiators by a supramolecular nanocapsule in aqueous solution. We demonstrate the remarkable stability of the initiators toward light and heat in the well-defined cavity shielded by the polyaromatic capsule shell. The incarcerated and stabilized initiators can be directly utilized for the radical polymerization of olefins on spontaneous release of the initiators from the capsule under the reaction conditions. Intrinsic properties of molecules can be altered on encapsulation within artificial or biological nanospaces [1] , [2] , [3] , [4] , [5] , [6] , [7] , [8] . Stabilization of highly reactive molecules in the confines of molecular capsules enabled the spectroscopic and even crystallographic observation of labile species such as cyclopolyenes [9] , [10] , benzyne [11] , peroxide [12] , phosphoniums [13] , oligosilanols [14] , iminiums [15] , hemiaminals [16] and white phosphorus [17] . The capsules function as protective, nanometre-sized containers and shield the guest molecules from external reagents, solvents, water and air. However, there are only a few reports on stabilizing reactive species toward light-triggered reactions through encapsulation [18] , [19] ; the majority of synthetic host frameworks are constructed from aliphatic or small aromatic subunits and are thus unable to shield bound guests from external light. Polyaromatic panels, composed of multiple, extended aromatic rings, effectively absorb ultraviolet (UV) light, with high extinction coefficients and thereby prevent the penetration of photons [20] , [21] . Therefore, we envisioned that a molecular capsule composed of polyaromatic frameworks could offer a new class of molecular flasks whereby the photo-reactivities of guest substrates can be manipulated through encapsulation. Here, we report the remarkable stability of radical initiators toward light and heat on encapsulation by supramolecular nanocapsule 1 ( Fig. 1a,b ). Furthermore, the incarcerated initiators retain their synthetic utility and can initiate the radical polymerization of olefins on release from the capsule, through equilibrium processes, under the reaction conditions. 2,2'-Azobisisobutyronitrile (AIBN) and its derivatives ( Fig. 1c ) are well-known and useful radical initiators for various polymer and organic syntheses on the small scale and are commonly employed in industry at the huge scale [22] , [23] . Azo-based radical initiators generate organic radical species irreversibly by releasing dinitrogen, triggered by photo or thermal stimuli. The initiators are so unstable due to the thermodynamic favorability of N 2 release that they should be stored in the dark at low temperature to prevent photochemical or thermal decomposition and accidental explosion. We reasoned that the stability of photochemically and thermally sensitive radical initiators, AIBN and its derivatives, could be enhanced on encapsulation by capsule 1 by the shielding effect of the polyaromatic frameworks. Supramolecular nanocapsule 1 provides a spherical cavity protected by eight anthracene panels ( Fig. 1b ) [24] , [25] , [26] . The capsule assembles from two Pd(II) ions and four bent bispyridine ligands 2 with two embedded anthracene rings in a quantitative yield and encapsulates neutral guest molecules with the size up to 1 nm, in which the guests are shaded from the outside by the closed polyaromatic shell. 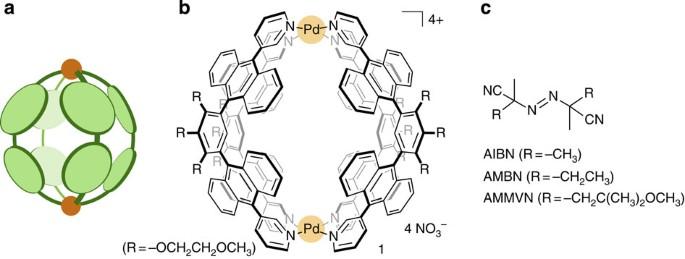Figure 1: Structure of a supramolecular nanocapsule and radical initiators. (a) Cartoon and (b) chemical structure of nanocapsule1and (c) radical initiators: AIBN, AMBN and AMMVN. Figure 1: Structure of a supramolecular nanocapsule and radical initiators. ( a ) Cartoon and ( b ) chemical structure of nanocapsule 1 and ( c ) radical initiators: AIBN, AMBN and AMMVN. Full size image Encapsulation of AIBN by capsule 1 Supramolecular capsule 1 spontaneously encapsulated one molecule of AIBN by hydrophobic interactions and the resultant inclusion complex was confirmed by nuclear magnetic resonance (NMR), mass spectrometry (MS) and X-ray crystallographic analyses. When AIBN (0.75 μmol) was suspended in a 9:1 D 2 O/CD 3 CN solution (0.5 ml) of capsule 1 (0.75 μmol) at room temperature, the 1:1 inclusion complex, 1 ⊃ AIBN, was formed quantitatively within 1 min ( Fig. 2a ). In the 1 H NMR spectrum, the methyl signal derived from AIBN was desymmetrized and observed at −1.95 and −1.81 p.p.m. with outstanding upfield shifts ( Δδ max =−3.65 p.p.m.) due to the encapsulation in the capsule with tightly wound anthracene panels ( Fig. 2b,c ). A slight shift of the inner phenylene signal ( H a ) also indicated the accommodation of AIBN in 1 . Quantitative formation of a 1:1 host–guest complex was demonstrated by 1 H NMR integration and electrospray ionization time-of-flight (ESI-TOF) MS analysis: prominent MS signals observed at m/z 900.7, 1,222.2 and 1,863.8 were assigned to [ 1 ⊃ AIBN— n· NO 3 − ] n + species ( n =4, 3 and 2, respectively; Fig. 2d ). Finally, pale-yellow single crystals were obtained by slow concentration of a H 2 O/CH 3 CN (9:1) solution of 1 ⊃ AIBN over 1 week. Crystallographic analysis of 1 ⊃ AIBN confirmed that the single AIBN guest molecule is shielded from the external environment by the anthracene panels of capsule 1 ( Fig. 2e,f ). The crystal structure also revealed that the enclathrated AIBN guest adopts an S-shaped trans configuration, where the CN groups point toward the Pd centres (where the CN-Pd distances are ~0.35 nm) in the cavity. Infrared (IR) spectroscopy suggested the existence of weak electrostatic interactions between the CN groups and the Pd ions. 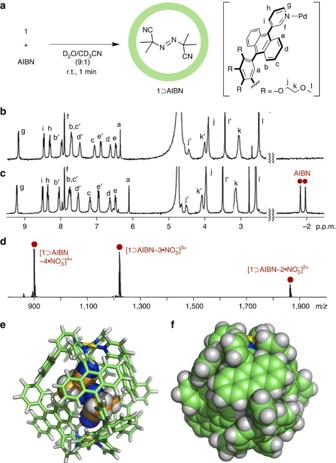Figure 2: Formation and characterization of capsule 1⊃AIBN. (a) Schematic representation of the encapsulation of AIBN within capsule1in aqueous solution.1H NMR spectra (400 MHz, room temperature, D2O/CD3CN (9/1)) of (b) capsule1and (c)1⊃AIBN. (d) ESI-TOF MS spectrum of1⊃AIBN. X-ray crystal structure of1⊃AIBN: (e) space-filling (for AIBN) and cylindrical (for1) representation and (f) space-filling representation (substituents and counterions are omitted for clarity). Figure 2: Formation and characterization of capsule 1 ⊃ AIBN. ( a ) Schematic representation of the encapsulation of AIBN within capsule 1 in aqueous solution. 1 H NMR spectra (400 MHz, room temperature, D 2 O/CD 3 CN (9/1)) of ( b ) capsule 1 and ( c ) 1 ⊃ AIBN. ( d ) ESI-TOF MS spectrum of 1 ⊃ AIBN. X-ray crystal structure of 1 ⊃ AIBN: ( e ) space-filling (for AIBN) and cylindrical (for 1 ) representation and ( f ) space-filling representation (substituents and counterions are omitted for clarity). Full size image Photostability of AIBN and its derivatives within capsule 1 The AIBN initiator was found to be stable toward UV light in the confines of capsule 1 . A solution of 1 ⊃ AIBN in D 2 O/CD 3 CN (1.5 mM) was irradiated for 10 h at room temperature, whereon 1 H NMR analysis revealed the AIBN molecule encapsulated within the capsule remained intact ( Fig. 3a,b ). Free AIBN, on the other hand, completely decomposed into tetramethylsuccinonitrile (TMSN) and other by-products under similar conditions ( λ irrad =360 nm for 10 h in CD 3 OD) in the absence of the capsule ( Fig. 3c,d ). Kinetic analysis of the decomposition revealed half-lives ( τ 1/2 ) of ≥690 and 1.8 h for the encapsulated AIBN and free AIBN, respectively ( Fig. 3e ). Thus AIBN is stabilized toward UV light by ≥380 times within the capsule (See Supplementary Table 1 ). We attribute the observed stability of enclathrated AIBN toward light to the optical shielding of the polyaromatic shell of capsule 1 ( Fig. 2f ). UV-visible spectrum of capsule 1 showed strong absorption bands ( ε =72,000 l mol −1 cm −1 at 380 nm) in the range of 300–450 nm due to the π–π* transitions of the embedded anthracene moieties. The bands fully occlude the weak absorption band of AIBN ( ε =14 l mol −1 cm −1 at 345 nm), illustrating that the encapsulated initiators are effectively shielded from UV light in the capsule. 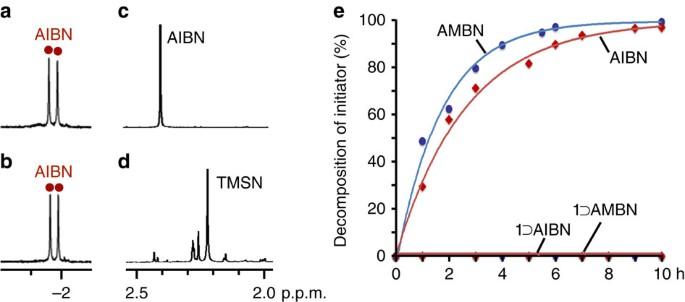Figure 3: Photostability of radical initiators AIBN and AMBN within/without capsule 1. 1H NMR spectra (400 MHz, room temperature) of1⊃AIBN (a) before and (b) after UV irradiation (λirrad=360 nm) in D2O/CD3CN (9/1) for 10 h and free AIBN (c) before and (d) after UV light irradiation (λirrad=360 nm) in CD3OD for 10 h. (e) Time course of the decomposition of AIBN and AMBN within/without1on UV irradiation (λirrad=360 nm) at room temperature. Figure 3: Photostability of radical initiators AIBN and AMBN within/without capsule 1. 1 H NMR spectra (400 MHz, room temperature) of 1 ⊃ AIBN ( a ) before and ( b ) after UV irradiation ( λ irrad =360 nm) in D 2 O/CD 3 CN (9/1) for 10 h and free AIBN ( c ) before and ( d ) after UV light irradiation ( λ irrad =360 nm) in CD 3 OD for 10 h. ( e ) Time course of the decomposition of AIBN and AMBN within/without 1 on UV irradiation ( λ irrad =360 nm) at room temperature. Full size image Similar to AIBN, the slightly larger radical initiator, 2,2'-azobis(2-methylbutyronitrile) (AMBN), was quantitatively encapsulated in capsule 1 and the resultant host–guest complex also displayed stability for UV light irradiation (See Supplementary Table 1 ). The τ 1/2 for the decomposition of AMBN within 1 was estimated to be over 690 h, indicating that the photostability is more than 580 times enhanced as compared with that of free AMBN ( Fig. 3e ). The even larger AIBN derivative, 2,2'-azobis(4-methoxy-2,4-dimethylvaleronitrile) (AMMVN) [27] was also encapsulated by capsule 1 . Although the diameter of the radical initiator (1.6 nm) is longer than that of the inner cavity of 1 (~1.0 nm), a single molecule of AMMVN entered the cavity of 1 in H 2 O/CH 3 CN solution, as confirmed by NMR and MS analyses ( Fig. 4a–c ). Host–guest complex 1 ⊃ AMMVN showed high stability against UV light: τ 1/2 values for the decomposition of AMMVN within and without 1 were 70 and 1.5 h, respectively ( Fig. 4d ). These results further demonstrate that capsule 1 can serves as a molecular container for safekeeping radical initiators under light. 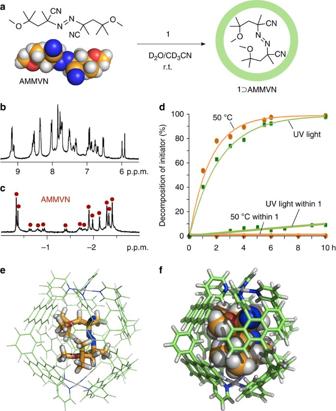Figure 4: Encapsulation, characterization and stabilization of AMMVN within capsule 1. (a) Schematic representation of the encapsulation of AMMVN within capsule1in aqueous solution.1H NMR spectra (400 MHz, room temperature, D2O/CD3CN (9/1)) of1⊃AMMVN in (b) the aromatic and (c) aliphatic regions. (d) Photostability (λirrad=360 nm, room temperature) and thermal stability (50 °C, dark) of AMMVN within/without1. X-ray crystal structure of1'⊃AMMVN: (e) stick (for1') and cylindrical (for AMMVN) and (f) cylindrical (for1') and space-filling (for AMMVN) representations (substituents and counterions are omitted for clarity). Figure 4: Encapsulation, characterization and stabilization of AMMVN within capsule 1. ( a ) Schematic representation of the encapsulation of AMMVN within capsule 1 in aqueous solution. 1 H NMR spectra (400 MHz, room temperature, D 2 O/CD 3 CN (9/1)) of 1 ⊃ AMMVN in ( b ) the aromatic and ( c ) aliphatic regions. ( d ) Photostability ( λ irrad =360 nm, room temperature) and thermal stability (50 °C, dark) of AMMVN within/without 1 . X-ray crystal structure of 1' ⊃ AMMVN: ( e ) stick (for 1' ) and cylindrical (for AMMVN) and ( f ) cylindrical (for 1' ) and space-filling (for AMMVN) representations (substituents and counterions are omitted for clarity). Full size image Thermal stability of AMMVN within capsule 1 Remarkably, in the polyaromatic shell of capsule 1 , AMMVN remained intact at room temperature for several weeks and on heating at 50 °C for over 10 h ( Fig. 4d ). AMMVN is one of the most thermally reactive initiators among reported AIBN derivatives and decomposition occurs even at room temperature (for example, τ 1/2 =10 h at 30 °C and τ 1/2 =1.1 h at 50 °C; Fig. 4d ). In the solid state, AMMVN completely decomposed at 50 °C (or under UV irradiation ( λ max =360 nm)) for 10 h, whereas AMMVN encapsulated by the capsule remained intact under the same conditions. This unusual thermal stability can be rationalized through the tight encapsulation of the large radical initiator by capsule 1 through hydrophobic interactions. Elongation of the N–C bonds ( Δd =0.05 nm) of AIBN and the derivatives along the reaction pathway is essential for the generation of the radical species through homolytic bond cleavage [28] . However, AMMVN fully fills the capsule cavity and thereby the formation of the lengthened transition state, with accompanying bond lengthening and volume expansion, should be energetically disfavored. X-ray crystallographic analysis of 1' ⊃ AMMVN (which is an analogue of 1 ⊃ AMMVN, where the Pd(II) ions are replaced by Pt(II) ions) revealed that the AMMVN guest occupies 64% of the cavity volume (~0.55 nm 3 ) by using VOIDOO program (See Supplementary Table 2 ) [29] . In the crystal structure, the encapsulated AMMVN adopts an otherwise labile C-shaped conformation arising from structural complementarity with the spherical cavity ( Fig. 4e,f ) [30] , [31] , [32] . Gas-phase calculations (DFT, B3LYP/6-31G* level) indicated the energy of the observed conformation of AMMVN is >60 kcal mol −1 higher than that of the optimized conformation without the capsule (See Supplementary Table 3 ). We hypothesize that a tight fit is essential for thermal stabilization. Host–guest complexes of the smaller AIBN and AMBN with 1 showed no increase in thermal stability relative to the free guests in organic solution: AIBN and AMBN completely decomposed at 65 °C for 48 h in free solution and even within host 1 . Interestingly, the thermal decomposition of AIBN within 1 gave rise to TMSN in quantitative yield, whereas that without 1 yielded a mixture of TMSN (~20%) and other by-products (~80%) under similar conditions. Thermal and photochemical polymerization of MMA Encapsulated 1 ⊃ AIBN and 1 ⊃ AMMVN retained reactivity as radical initiators for standard radical polymerization reactions in organic solution through release of the initiators from the capsule ( Fig. 5 ). The initiators are bound in the capsule by non-covalent hydrophobic interactions and thus subject to reversible binding processes under equilibrium. A pale-yellow powder of 1 ⊃ AIBN was obtained from the aqueous solution on solvent evaporation. A toluene solution (100 μl) of methyl methacrylate (MMA; 1.9 mmol) and 1 ⊃ AIBN (0.75 μmol, [MMA]/[ 1 ⊃ AIBN]=2,533) was then heated at 80 °C for 24 h and the resultant solution solidified due to poly(methylmethacrylate) (PMMA) formation. The polymer was isolated by the addition of a CH 2 Cl 2 solution of the reaction mixtures into CH 3 OH and was washed with CH 3 OH. The yield and average molecular weight ( M n ) of the obtained PMMA were determined to be 84% and 1.08 × 10 5 , respectively. These results are comparable to PMMAs prepared by the use of free AIBN (0.75 μmol) under similar conditions (See Supplementary Table 4 ). The molecular weight distribution of the obtained polymers ( M w / M n =2.8) was insensitive to the existence of the capsule. Photopolymerization of MMA in toluene solution containing 1 ⊃ AIBN gave rise to similar PMMA (86% yield, M w =1.61 × 10 5 ) on irradiation by a Xe lamp (150 W) for 24 h at room temperature. The 1 ⊃ AMMVN initiator complex also successfully initiated the thermal and photochemical polymerizations of MMA (See Supplementary Table 4 ). 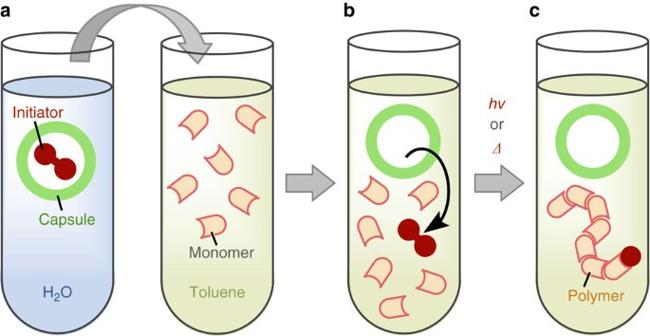Figure 5: Schematic representation of olefin polymerization with capsule1containing a radial initiator. (a) Addition of the capsulated initiator to an organic solution of monomers. (b) Spontaneous release of the initiator from the capsule. (c) Polymerization of the monomers initiated by the initiator on photo or thermal stimuli. Figure 5: Schematic representation of olefin polymerization with capsule 1 containing a radial initiator. ( a ) Addition of the capsulated initiator to an organic solution of monomers. ( b ) Spontaneous release of the initiator from the capsule. ( c ) Polymerization of the monomers initiated by the initiator on photo or thermal stimuli. Full size image In this study, we successfully controlled the stabilities of well-known and widely used radical initiators, AIBN and its derivatives, toward light through encapsulation within a supramolecular nanocapsule with polyaromatic frameworks. The encapsulation process occurs quantitatively by hydrophobic host–guest interactions in less than one minute in aqueous solution at room temperature. The encapsulated initiators in the capsule were significantly stabilized against light irradiation (up to 580 times) due to optical filtering by the polyaromatic frameworks. Furthermore, the thermal stabilization of large AIBN derivative (645 times) was accomplished through encapsulation in tight fitting molecular capsule of complementary size and shape. The safely stored initiators could be used for usual olefin polymerization in organic solvent through spontaneous release of the initiators. We emphasize that well-defined, constrictive nanospaces enclosed by a self-assembled polyaromatic shell are ideal for manipulating both the photochemical and thermal reactivity of encapsulated guest molecules. General NMR: Bruker AVANCE-400 (400 MHz), ESI-TOF MS: Bruker micrOTOF II, FT-IR: JASCO FT/IR-4200, UV–vis: JASCO V-670DS, UV light irradiation: Soma Kogaku Xe lamp (150 W) at a distance of 7.0 cm, X-ray: APEXII DUO/CCD diffractometer, GPC: TOSO HLC-8120GPC (40 °C, 0.5 ml min −1 ) with Shodex SB-802.5 HQ and SB-806 M HQ columns. Solvents and reagents: TCI Co., Ltd., WAKO Pure Chemical Industries Ltd., KANTO kagaku KANTO CHEMICAL CO., INC., Sigma-Aldrich Co. and Cambridge Isotope Laboratories, Inc. Ligand 2 and Pd-capsule 1 (See Supplementary Methods and Supplementary Figs 1–3 ) were synthesized according to previously reported procedures [24] , [33] . Formation of 1 ⊃ AIBN Pd-capsule 1 (2.8 mg, 0.75 μmol), AIBN (0.12 mg, 0.75 μmol), D 2 O (0.45 ml) and CD 3 CN (0.05 ml) were added to a brown glass test tube. The mixture was stirred at room temperature for 1 min. The quantitative formation of a 1 ⊃ AIBN complex was confirmed by NMR and ESI-TOF MS analyses (See Supplementary Figs 4–7 ). Pale-yellow single crystals suitable for X-ray crystallographic analysis were obtained by slow concentration of a H 2 O(+NaCl)/CH 3 CN (9:1) solution of 1 ⊃ AIBN at room temperature over 1 week (See Supplementary Fig. 8 and Supplementary Table 5 ). Similarly, a 1 ⊃ AMBN complex was prepared in quantitative yield (See Supplementary Methods and Supplementary Figs 9–12 ). 1 H NMR (400 MHz, D 2 O:CD 3 CN=9:1, room temperature): δ −1.95 (s, 6H, AIBN), −1.81 (s, 6H, AIBN), 2.56 (s, 24H), 3.21 (m, 16H), 3.49 (s, 12H), 3.84–4.15 (m, 24H), 4.41–4.67 (m, 8H), 6.08 (s, 4H), 6.46 (d, J =8.4 Hz, 8H), 6.61 (dd, J =7.2, 8.4 Hz, 8H), 6.93 (d, J =8.4 Hz, 8H), 7.17 (dd, J =7.2, 8.4 Hz, 8H), 7.51 (dd, J =7.2, 8.4 Hz, 8H), 7.72–7.77 (m, 16H), 7.89 (s, 8H), 8.04 (d, J =8.4 Hz, 8H), 8.35 (dd, J =5.6, 7.6 Hz, 8H), 8.49 (d, J =7.6 Hz, 8H), 9.20 (d, J =5.6 Hz, 8H). IR (KBr, cm −1 ): 3,062, 2,983, 2,929, 2,882, 2,817, 2,239, 1,945, 1,637, 1,384, 1,194, 1,125, 1,104, 1,065, 1,029, 943, 768, 706, 671, 644. ESI-TOF MS (H 2 O): m/z 1,863.8 [ 1 ⊃ AIBN—2NO 3 − ] 2+ , 1,222.2 [ 1 ⊃ AIBN—3NO 3 − ] 3+ , 900.7 [ 1 ⊃ AIBN—4NO 3 − ] 4+ . Formation of 1 ⊃ AMMVN Pd-capsule 1 (2.8 mg, 0.75 μmol), AMMVN (0.23 mg, 0.75 μmol), D 2 O (0.45 ml) and CD 3 CN (0.05 ml) were added to a brown glass test tube. The mixture was stirred at room temperature for 1 min. The quantitative formation of a 1 ⊃ AMMVN complex was confirmed by NMR and ESI-TOF MS analyses (See Supplementary Figs 13–16 ). Pale-yellow single crystals suitable for X-ray crystallographic analysis were obtained by slow concentration of a H 2 O/CH 3 CN (9:1) solution of 1′ ⊃ AMMVN at room temperature over 1 week (See Supplementary Methods and Supplementary Figs 17–21 and Supplementary Table 6 ). 1 H NMR (400 MHz, D 2 O:CD 3 CN=9:1, room temperature): δ −2.39 (s, AMMVN), −2.31 (s, AMMVN), −2.27 (s, AMMVN), −2.11 (s, AMMVN), −1.97 (s, AMMVN), −1.89 (s, AMMVN), −1.70 (br, AMMVN), −1.38 (d, J =14.0 Hz, AMMVN), −0.90 (d, J =14.0 Hz, AMMVN), −0.80 (d, J =14.0 Hz, AMMVN), −0.61 (d, J =14.0 Hz, AMMVN), −0.35 (s, AMMVN), −0.31 (s, AMMVN), 2.61–2.65 (m, 24H), 3.02–3.32 (m, 16H), 3.54 (d-like, 12H), 3.86–4.28 (m, 24H), 4.28–4.69 (m, 8H), 5.94–6.02 (m, 4H), 6.56 (d, J =8.8 Hz, 4H), 6.71–7.02 (m, 20H), 7.33–7.50 (m, 8H), 7.54 (dd, J =7.2, 8.8 Hz, 8H), 7.74–7.81 (m, 16H), 7.87 (s, 8H), 8.05 (d, J =8.8 Hz, 8H), 8.39 (br, 8H), 8.56–8.61 (m, 8H), 9.14–9.21 (m, 8H). IR (KBr, cm −1 ): 3,063, 2,978, 2,933, 2,883, 2,822, 2,239, 1,950, 1,839, 1,655, 1,384, 1,242, 1,195, 1,065, 1,029, 942, 769, 706, 670, 611. ESI-TOF MS (H 2 O): m/z 1,936.6 [ 1 ⊃ AMMVN—2NO 3 − ] 2+ , 1,270.4 [ 1 ⊃ AMMVN—3NO 3 − ] 3+ , 937.1 [ 1 ⊃ AMMVN—4NO 3 − ] 4+ . Photostability of AIBN within 1 1 ⊃ AIBN complex (2.9 mg, 0.75 μmol), D 2 O (0.45 ml) and CD 3 CN (0.05 ml) were added to a NMR tube under N 2 . 1 H NMR spectrum of the solution was measured before and after UV light irradiation (360 nm) at room temperature for 10 h (See Supplementary Figs 22–24 ). Similarly, the photostability of AMBN within 1 was studied (See Supplementary Figs 24–26 ). Photostability of AMMVN within 1 1 ⊃ AMMVN complex (3.0 mg, 0.75 μmol), D 2 O (0.45 ml) and CD 3 CN (0.05 ml) were added to a NMR tube under N 2 . 1 H NMR spectrum of the solution was measured before and after UV light irradiation (360 nm) at room temperature for 10 h (See Supplementary Figs 24 and 27–29 ). Photostability of AMMVN within 1 in the solid state was also studied (See Supplementary Fig. 30 ). Thermal stability of AIBN within 1 1 ⊃ AIBN complex (2.9 mg, 0.75 μmol), D 2 O (0.45 ml) and CD 3 CN (0.05 ml) were added to a NMR tube. 1 H NMR spectrum of the solution was measured before and after heating at 65 °C for 2 days (See Supplementary Figs 24 and 31 ). Similarly, the thermal stability of AMBN within 1 was studied (See Supplementary Methods and Supplementary Figs 24 and 32 ). Thermal stability of AMMVN within 1 1 ⊃ AMMVN complex (3.0 mg, 0.75 μmol), D 2 O (0.45 ml) and CD 3 CN (0.05 ml) were added to a NMR tube. 1 H NMR spectrum of the solution was measured before and after heating at 50 °C for 33 h (See Supplementary Figs 24, 33 and 34 ). Thermal stability of AMMVN within 1 in the solid state was also studied (See Supplementary Fig. 35 ). Thermal polymerization of MMA by AIBN or 1 ⊃ AIBN AIBN (0.12 mg, 0.75 μmol) or 1 ⊃ AIBN (2.9 mg, 0.75 μmol), MMA (0.2 ml, 1.9 mmol) and toluene (0.1 ml) were added to a 5 ml Schlenk flask under N 2 . The mixture was heated at 80 °C for 24 h. The crude product was dissolved to CH 2 Cl 2 (5 ml) and then the resultant solution was poured into methanol (50 ml). The precipitate was collected, washed with methanol and dried under reduced pressure to afford PMMA as a white solid (166 mg (88% yield) from AIBN initiator, 159 mg (84% yield) from 1 ⊃ AIBN initiator; See Supplementary Figs 36 and 37 and Supplementary Table 4 ). Thermal polymerization of MMA by 1 ⊃ AMMVN also afforded PMMA (See Supplementary Methods and Supplementary Fig. 38 and Supplementary Table 4 ). Photopolymerization of MMA by AIBN or 1 ⊃ AIBN AIBN (0.12 mg, 0.75 μmol) or 1 ⊃ AIBN (2.9 mg, 0.75 μmol), MMA (0.2 ml, 1.9 mmol) and toluene (0.05 ml) were added to a 5 ml Schlenk flask under N 2 . The mixture was irradiated with a UV lamp (no cut filter) at room temperature for 24 h. The crude product was dissolved to CH 2 Cl 2 (5 ml) and then the resultant solution was poured into methanol (50 ml). The precipitate was collected, washed with methanol and dried under reduced pressure to afford PMMA as a white solid (164 mg (87% yield) from AIBN initiator, 162 mg (86% yield) from 1 ⊃ AIBN initiator; See Supplementary Fig. 39 and Supplementary Table 4 ). Photopolymerization of MMA by 1 ⊃ AMMVN also afforded PMMA (See Supplementary Methods and Supplementary Fig. 40 and Supplementary Table 4 ). Accession codes: CCDC-990095 and 990110 contain the supplementary crystallographic data for the structures reported in this article. These data can be obtained free of charge from The Cambridge Crystallographic Data Centre (CCDC) via www.ccdc.cam.ac.uk/data_request/cif How to cite this article: Yamashina, M. et al . Safe storage of radical initiators within a polyaromatic nanocapsule. Nat. Commun. 5:4662 doi: 10.1038/ncomms5662 (2014).